Porous boron nitride nanosheets for effective water cleaning Effective removal of oils, organic solvents and dyes from water is of significant, global importance for environmental and water source protection. Advanced sorbent materials with excellent sorption capacity need to be developed. Here we report porous boron nitride nanosheets with very high specific surface area that exhibit excellent sorption performances for a wide range of oils, solvents and dyes. The nanostructured material absorbs up to 33 times its own weight in oils and organic solvents while repelling water. The saturated boron nitride nanosheets can be readily cleaned for reuse by burning or heating in air because of their strong resistance to oxidation. This easy recyclability further demonstrates the potential of porous boron nitride nanosheets for water purification and treatment. Oil spillage, organic solvents and dyes discharged by the textile, paper and tannery industries are primary pollutants of water sources [1] , [2] . Sorption is an efficient way to clean-up water but common absorbents, including activated carbon [3] , zeolites [4] , and natural fibers [5] , suffer from low separation selectivity and low absorption capacity. A number of advanced materials [6] , [7] , [8] , [9] have been developed and suggested to overcome these principal drawbacks, but they still show unsatisfactory regeneration and cycling ability. Indeed, besides good absorbing properties in terms of capacity and kinetics, the desired absorbent materials should exhibit light weight for high gravimetric capacity, easy separation from cleaned water and easy cleaning for long-term cycling. Boron nitride (BN) nanosheets, so-called ‘white graphene’, consist of a few layers of hexagonal BN planes and have unique properties compared with graphene, including a wide energy band gap, electrical insulation, ultraviolet (UV) photoluminescence, high thermal conductivity and stability, and high resistance to oxidation and chemical inertness [10] , [11] , [12] , [13] . In addition, the polarity of BN bonds and the high surface area of h -BN-related nanostructures provide good adsorption properties of various substances ranging from organic pollutants [14] to hydrogen [15] . As BN is composed of light elements, it promises absorbents of high uptake gravimetric capacity. Its high chemical and thermal stability also suggests that recycling could be easily achieved. Nanostructured BN is therefore an ideal candidate as an absorbent material [16] , [17] . Here we report the development of a layered BN nanomaterial combining highly porous and nanosheet structures with superior performance in the whole scope of the absorbing process, including capacity, kinetics, recovery, regeneration and cycling. The specific surface area of these porous BN nanosheets is among the highest reported to date (1,427 m 2 g −1 ) ( [18] ) and the material shows excellent sorption performances for a wide range of oils, solvents and dyes, with mass uptakes reaching 3,300%, due to a combination of superhydrophobicity, porosity and swelling ability. Furthermore, the saturated material can be cleaned for reuse by simply washing, burning or heating in air because of its strong resistance to oxidation. These easy recycling routes further demonstrate the great potential of porous BN nanosheets for water purification and treatment. Synthesis We developed a synthesis process of porous BN nanosheets relying on a dynamic templating approach. Side products of the condensation of the solid framework evolve as nanobubles that act as fugitive templates of the final porous structure [19] . Briefly, a homogeneous mixture of boron trioxide and guanidine hydrochloride as, respectively, boron and nitrogen sources were heated in a tube furnace at 1,100 °C for 2 h under H 2 /N 2 (15 vol% hydrogen) gas flow to yield a white product. X-ray powder diffraction (XRD, Supplementary Fig. S1 ) and X-ray photoelectron spectroscopy (XPS, Supplementary Fig. S2 ) analyses show typical crystalline structure related to h -BN and clear BN bonding. Scanning electron microscopy (SEM, Fig. 1a ), transmission electron microscopy (TEM, Fig. 1c ) and atomic force microscopy (AFM, Fig. 1e inserts) examinations reveal that the BN nanosheets have many holes of diameters ranging from 20 to 100 nm, which are created by gas bubbles during the formation process. It is well known that guanidine hydrochloride decomposes at high temperature by releasing a number of gaseous species including N 2 , HCl and NH 3 ( [20] ). The selected-area electron diffraction ( Fig. 1c insert) pattern shows two characteristic diffraction rings ((002) and (100)) of layered BN related to h -BN in consistency with the XRD results. The high-resolution TEM ( Fig. 1d ) image shows three parallel fringes at the edge region of a sheet. The d -spacing of 0.34 nm is close to the (002) plane interdistance and suggests three stacked BN layers in the nanosheet. This is consistent with the thickness of about 1.1 nm evaluated by the AFM line-scan profile ( Fig. 1e insert). Highly porous structure can be seen clearly from the TEM and AFM images in Fig. 1 . 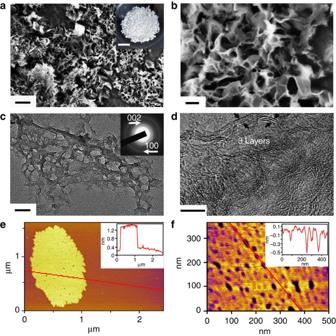Figure 1: Nanostructure of porous BN nanosheets. (a) Low-magnification SEM image of the porous BN nanosheets. Scale bar, 2 μm. The inset shows the typical white powder obtained after synthesis. Scale bar, 1 cm. (b) High-magnification SEM image revealing the porous nanosheet structure. Scale bar, 200 nm. (c) TEM image of a single nanosheet showing holes on the nanosheet, inserted selected-area electron diffraction pattern indicating a layered BN structure. Scale bar, 50 nm. (d) High-resolution TEM image of the edge folding of a nanosheet with three BN layer domains highlighted by black arrows. Scale bar, 5 nm. (e) AFM image of a nanosheet and the inserted height profiles showing typical size and thickness of a single nanosheet. (f) High-magnification AFM image and the corresponding height profiles inserted. The porous structure can be seen clearly. Figure 1: Nanostructure of porous BN nanosheets. ( a ) Low-magnification SEM image of the porous BN nanosheets. Scale bar, 2 μm. The inset shows the typical white powder obtained after synthesis. Scale bar, 1 cm. ( b ) High-magnification SEM image revealing the porous nanosheet structure. Scale bar, 200 nm. ( c ) TEM image of a single nanosheet showing holes on the nanosheet, inserted selected-area electron diffraction pattern indicating a layered BN structure. Scale bar, 50 nm. ( d ) High-resolution TEM image of the edge folding of a nanosheet with three BN layer domains highlighted by black arrows. Scale bar, 5 nm. ( e ) AFM image of a nanosheet and the inserted height profiles showing typical size and thickness of a single nanosheet. ( f ) High-magnification AFM image and the corresponding height profiles inserted. The porous structure can be seen clearly. Full size image The N 2 sorption isotherm of the porous BN nanosheets ( Supplementary Fig. S3a ) can be categorized as type II based on the IUPAC classification, type H3 hysteresis loop in the relative pressure range of 0.4–1.0 indicating the presence of mesopores with a diameter below 20 nm. The abrupt closure at a relative pressure of ca. 0.42 suggests the presence of slit-shaped pores, in accordance with the sheet-like shape of the nanostructures. The total pore volume is 1.09 cm 3 g −1 . Calculation according to the BET model gives a specific surface area of 1,427 m 2 g −1 . BJH calculations give a pore size distribution ranging from 20 to 100 nm. The narrowness of the hysteresis in the isothermal curve suggests that the majority of pores belong to the family of macropores, with a diameter higher than 50 nm. This is confirmed by SEM, TEM and AFM images ( Fig. 1 ). The high surface area comes from both the intra-sheet holes and the inter-sheet space, the latter giving rise to slit-shaped porosity. Such a high surface area is among the highest ones reported so far in any BN material [18] . Porous BN nanosheets are superhydrophobic with a contact angle of about 165° ( Supplementary Fig. S3c ). The Fourier transform infrared (FTIR) spectrum ( Supplementary Fig. S4 ) exhibits bands in the 2,950–2,800 cm −1 region, indicating the presence of CH x -containing species. These adsorbed molecules originate from ambient atmosphere and might be the cause of hydrophobicity, as proposed by Boinovich et al . [21] for BN nanotubes. The higher contact angle of porous nanosheets shows an increased hydrophobicity over the non-porous ones prepared by a similar method [22] ( Supplementary Fig. S3b,c ), which should be contributed by the rough surface nanostructuring as highlighted by the SEM pictures in Fig. 1a . It has been reported that the hydrophobicity of an already hydrophobic material can be increased by structuring its surface at the nanometre scale [23] . Therefore, the hydrophobicity of porous BN nanosheets originates primarily from adsorption of organics from ambient atmosphere, which is then exacerbated into superhydrophobicity by the surface nanostructuring, the so-called ‘Lotus effect’ [24] , [25] . Superhydrophobicity allows the porous BN nanosheets to float on the water surface and are therefore easy to be collected. Removal of oil and organic solvent from water Porous BN nanosheets exhibit excellent absorbencies for oils and organic solvents. 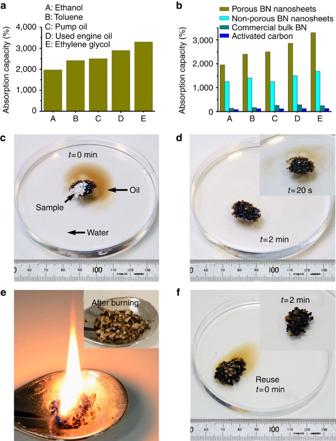Figure 2: Oils and organic solutions absorption properties. (a) Gravimetric absorption capacities of the porous nanosheets for five organic solvents and oils. (b) Comparison of the absorption capacities of the porous BN nanosheets with non-porous BN nanosheets, commercial bulk BN particles and activated carbon. (c) Photograph of the set-up for oil absorption tests with white porous BN nanosheets. (d) Photograph of porous BN nanosheets saturated with oil after 2 min of absorption, inset showing the absorption process after 20 s. (e) Photograph of burning oil-saturated porous BN nanosheets in air for cleaning purpose, inset showing the colour change after burning. (f) Photograph of the cleaned nanosheets for second oil absorption test, inset showing the absorption result after 2 min. Figure 2 a shows the uptakes of ethanol, toluene, pump oil, used engine oil and ethylene glycol with values ranging from 2,000 to 3,300 wt%. The porous BN nanosheets absorb up to 33 times their own weight of ethylene glycol and 29 times of used engine oil. Although not the highest one ever reported [26] , these uptakes are much higher than those of commercial activated carbon and BN particles ( Fig. 2b ), as well as most of the common absorbents and other recent refined materials, including graphene capsules [6] , collagen nanocomposites [7] , polyurethane sponge [8] , polyurethane and iron oxide composites [9] , MnO 2 nanowires [27] , and graphene hydrogels [28] . When non-porous BN nanosheets are tested under the same conditions, the absorbencies are decreased by half, indicating essential performance enhancement of porosity. The different steps of the absorption process of used engine oil are illustrated in Fig. 2c . Once the starting white nanosheets are dropped on the oil–water surface they immediately absorb the brown oil and become dark brown. This process is very fast ( Fig. 2d , inset at 20 s and Supplementary Movie 1 ); after just 2 min, all oil has been taken up by the nanosheets with a capacity of 2,900 wt%. The saturated nanosheets still float on the cleaned water surface and are therefore easy to be removed. Importantly, the material can be reused several times by directly burning it in air to remove the absorbed organics from the porous BN nanosheets ( Fig. 2e ), as used for other carbon sorbents [28] , [29] , [30] . Oil can be taken up again at least five times with a slight decrease in capacity ( Supplementary Fig. S5 : 2,500% at the first cycle, 1,800 wt% after five cycles for pump oil). Moreover, solvent extraction can be used as an alternative cleaning method to avoid the evolution of potentially harmful gases from burning oil; washing with organic solvents such as ethanol or petroleum ether enables recovery of the initial absorption capacity of porous BN nanosheets ( Supplementary Fig. S6 ). FTIR analysis ( Supplementary Fig. S4 ) reveals the presence of carbonaceous moieties in the burned porous BN nanosheets, which should be responsible to the remaining light colour ( Fig. 2f ), the slightly reduced efficiency, the slightly reduced water contact angle (143° after the first cycle) and partially blocked pores. The nanosheets can be cleaned completely by heating in a furnace at 600 °C for 2 h in air to almost regenerate all original properties ( Supplementary Figs S4, S5 and S7 ). The XRD ( Fig. 3a ) and TEM ( Supplementary Fig. S8 ) analyses performed on the calcined samples show that the crystallite size and the porosity are maintained after regeneration. This point is in stark contrast to other carbon-based materials and polymer-based sorbents that have higher initial capacities, but cannot stand such harsh conditions and therefore can only be used several times before porosity is completely filled by carbonaceous matter [29] , [30] . Figure 2: Oils and organic solutions absorption properties. ( a ) Gravimetric absorption capacities of the porous nanosheets for five organic solvents and oils. ( b ) Comparison of the absorption capacities of the porous BN nanosheets with non-porous BN nanosheets, commercial bulk BN particles and activated carbon. ( c ) Photograph of the set-up for oil absorption tests with white porous BN nanosheets. ( d ) Photograph of porous BN nanosheets saturated with oil after 2 min of absorption, inset showing the absorption process after 20 s. ( e ) Photograph of burning oil-saturated porous BN nanosheets in air for cleaning purpose, inset showing the colour change after burning. ( f ) Photograph of the cleaned nanosheets for second oil absorption test, inset showing the absorption result after 2 min. 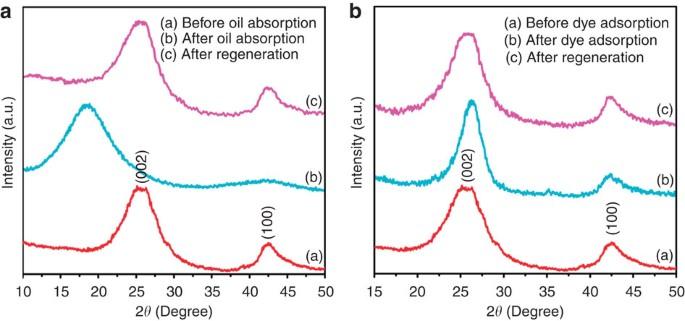Figure 3: Structural evolutions of porous BN nanosheets. XRD patterns of porous BN nanosheets during (a, left) used engine oil removal: before absorption (a), after absorption (b), after regeneration at 600 °C in air (c), and (b, right) congo red removal: before adsorption (a), after adsorption (b), after regeneration at 400 °C in air (c). Full size image Figure 3: Structural evolutions of porous BN nanosheets. XRD patterns of porous BN nanosheets during ( a , left) used engine oil removal: before absorption ( a ), after absorption ( b ), after regeneration at 600 °C in air ( c ), and ( b , right) congo red removal: before adsorption ( a ), after adsorption ( b ), after regeneration at 400 °C in air ( c ). Full size image Removal of dye from water Congo red (CR), an anionic dye, is considered as a primary toxic pollutant in water resources [31] . UV–visible (UV–vis) absorption spectroscopy was used at the maximum absorption wavelength of CR (496 nm) to estimate the adsorption kinetics from 10 mg of layered BN nanosheets in a 130 mg l −1 aqueous CR solution ( Fig. 4a ). After 60 min, the CR characteristic band became too weak to be observed, suggesting high efficiency for CR removal. 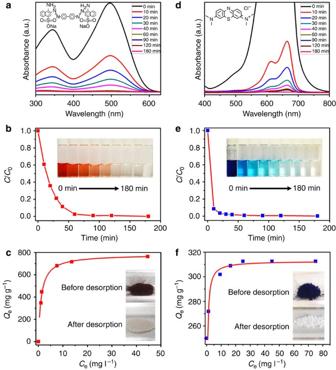Figure 4: Dyes adsorption properties. (a,d) UV–vis absorption spectra of the aqueous solutions of CR (130 mg l−1, 25 ml) and MB (110 mg l−1, 25 ml), respectively, in the presence of porous BN nanosheets at different intervals. The insets show the molecular structures of CR and MB, respectively. (b,e) Adsorption rates of CR and MB on porous BN nanosheets, respectively. The insets show the corresponding photographs. (c,f) Adsorption isotherms of CR and MB on porous BN nanosheets, respectively.Qe(mg g−1) is the amount of dyes adsorbed at equilibrium,Ce(mg l−1) is the equilibrium solute concentration. The insets present the photographs of the BN porous nanosheets with CR and MB composites before (upper) and after (bottom) recovering by heating at 400 °C for 2 h, respectively. Figure 4a show that about 99% of CR can be removed from water within 180 min at room temperature. The adsorption isotherm ( Fig. 4c ) fitted by the Langmuir model gives a maximum adsorption capacity Q m of 782 mg g −1 , corresponding to complete monolayer coverage. This capacity is significantly higher than those from most adsorbent nanomaterials reported previously [31] , [32] , [33] , [34] . The versatility of porous BN nanosheets for targeting a wide range of organic wastes has been assessed by testing other dyes with opposite charges commonly used in the textile industry, such as the cationic dyes methylene blue (MB) ( Fig. 4d–f ) and basic yellow 1 (BY) ( Supplementary Fig. S9 ). The maximum adsorption capacities of MB and BY are 313 and 556 mg g −1 , respectively. These values are greater than those reported for BN nanocarpets and BN hollow spheres [14] , [35] . Furthermore, the adsorbed dyes can be easily removed from the collected porous BN nanosheets by simply heating at 400 °C in air for 2 h (inserts in Fig. 4c ). The BN adsorbents are highly stable ( Fig. 3b ) and can be reused for several cycles without losing activity. Figure 4: Dyes adsorption properties. ( a , d ) UV–vis absorption spectra of the aqueous solutions of CR (130 mg l −1 , 25 ml) and MB (110 mg l −1 , 25 ml), respectively, in the presence of porous BN nanosheets at different intervals. The insets show the molecular structures of CR and MB, respectively. ( b , e ) Adsorption rates of CR and MB on porous BN nanosheets, respectively. The insets show the corresponding photographs. ( c , f ) Adsorption isotherms of CR and MB on porous BN nanosheets, respectively. Q e (mg g −1 ) is the amount of dyes adsorbed at equilibrium, C e (mg l −1 ) is the equilibrium solute concentration. The insets present the photographs of the BN porous nanosheets with CR and MB composites before (upper) and after (bottom) recovering by heating at 400 °C for 2 h, respectively. Full size image Both porous and non-porous [22] BN nanosheets show much higher absorbencies of oils than commercial bulk BN particles ( Fig. 2b ). This indicates that the nanosheet structure enhances the absorption capacity. In addition, the porous nanosheets exhibit a double capacity compared with non-porous nanosheets, suggesting the important role of intra-sheet porosity. XRD measurements were performed to assess the mechanism of sorption for oils ( Fig. 3a and Supplementary Fig. S10 ), ethanol ( Supplementary Fig. S11 ) and dyes ( Fig. 3b ) with both porous and non-porous nanosheets. For oil-saturated (for example, used engine oil) porous and non-porous BN nanosheets, a clear shift of the (002) diffraction peak to low angles is observed. This indicates that the interdistance between the (002) basal planes can increase by 37% from 0.35 nm to 0.48 nm through intercalation of the organic molecules in the inter-layer space. In contrast, the (002) peak of commercial bulk BN particles does not change ( Supplementary Fig. S12 ), which is consistent with the low oil sorption. Ethanol sorption leads to a smaller expansion of d (002) by 17%, which might be due to the alcohol hydrophilicity and the fast solvent evaporation during the slow XRD measurement. The increase in the inter-layer distance during absorption highlights the ability of the nanostructures to accommodate structural distortions and to swell while the bulk BN particles cannot stand such high strains. Therefore, the intercalation of molecules in the inter-layer space contributes to the uptake increase of the nanosheets. Indeed, nanosheet swelling provides additional capacity than expected from the porosity assessed by N 2 sorption. The sorption properties of porous BN nanosheets for oils and organic solvents can then be ascribed to (1) adsorption (surface effect) of molecules on the hydrophobic BN nanosheet surface; (2) capillarity effects for filling of the holes inside the nanosheets and the space between the sheets; (3) intercalation of molecules in the inter-layer space of the BN nanosheets. In brief, BN nanosheets show superior uptake of oils compared with commercial bulk BN particles and other common sorbents because of two reasons. First, the nanosheets can accommodate higher strains and faster molecular diffusion, thus enabling swelling. Second, their higher surface area and porosity ensure high uptake by adsorption and pore filling. In addition, because the inter-layer expansion is identical for porous and non-porous nanosheets ( Supplementary Figs S10 and S11 ), the increased capacity for the porous nanosheets compared with the non-porous ones is primarily due to the adsorption and pore-filling processes exacerbated by the higher surface area and pore volume. Contrary to oils sorption, there is no evidence of swelling when dyes are taken up ( Fig. 3b ). The holes inside the nanosheets and the space between the BN layers are mostly hydrophobic, as shown by the range of non-aqueous solvents that are absorbed with high uptakes. Capillarity effects in the hydrophobic sheets can then only take place with hydrophobic liquids, such as oils. Dyes are either at solid state in their pure form or as dilutes in hydrophilic (aqueous) solutions and cannot contribute to swelling of the nanosheets as a consequence of capillarity filling. Dyes sorption then only relies on the surface effect (adsorption of molecules on the hydrophobic BN nanosheet surface), which induces a lower capacity compared with oils and organic solvents. Nevertheless, the dyes sorption capacity of the porous BN nanosheets is still higher than those of most common commercial and state-of-the-art sorbents [14] , [31] , [32] , [33] , [34] , [35] , mainly because of their higher specific surface area. In addition, a large number of unsaturated atoms along the edges of the nanosheets and pores are chemically more reactive and might be stronger adsorption sites for organic molecules such as dyes [36] . In summary, highly porous BN nanosheets have been synthesised using a thermal treatment process without the use of any catalyst and ex situ template. The obtained porous BN nanosheets have a very high specific surface area as compared with other BN materials. They show superhydrophobicity, high selective absorption and adsorption capacities for oils, organic solvents and dyes, and thus can be used to clean contaminated water. These porous BN nanosheets can be reused many times for environmental remediation through regeneration upon burning or heating in air because of their high resistance to oxidation. All these features make these porous nanosheets suitable for a wide range of applications in water purification and treatment. Synthesis In a typical synthesis, 4 mmol (0.28 g) of boron trioxide and 20 mmol (1.95 g) of guanidine hydrochloride were mixed in 20 ml methanol to form a clear, colourless solution. After 24 h of fast stirring, a white crystalline powder (a complex between the boron trioxide and guanidine chloride) was formed. The crystalline powders were loaded into a quartz boat and then heated to 1,100 °C at a rate of 10 °C min −1 and the sample was kept at 1,100 °C for 2 h under a nitrogen—15% hydrogen gas flow to ensure a full nitridation. White porous BN nanosheets were produced with a yield of 50 mol% versus boron precursor. Materials characterisation X-ray diffraction patterns of the samples were collected using a Panalytical X’Pert PRO diffraction system with a Cu Kα radiation. The XPS spectra were obtained on an ESCALab MKII X-ray photoelectron spectrometer using non-monochromatised Mg-K a X-ray as the excitation source. The sample structure and morphology were studied using a JEOL 2100 TEM and a Zeiss Supra 55 VP SEM. The AFM measurements were performed on a Cypher atomic force microscope. Contact angle measurements were made by a contact angle goniometer (CAM101, KSV). Nitrogen adsorption and desorption isotherms were obtained using a Tristar 3000 apparatus at 77 K. The UV–vis absorption spectra were collected on a Cary 5000 spectrophotometer. FTIR spectra were obtained with a Nicolet 7199 FTIR spectrometer. Oil and organic solvent removal tests Five different kinds of organic solvents and oils with different densities, including ethanol, toluene, ethylene glycol, pump oil and used engine oil, were used in this study. The absorption capacity values, W (wt/wt) %, were obtained by measuring the mass of the dry porous BN nanosheets, and then the mass after oil/solvent absorption. The samples were left submerged in the solvents or oils fully for overnight to ensure full saturation was obtained before weighing. Weight measurements were done rapidly to avoid evaporation of absorbed solvents or oils. The non-porous nanosheets and activated carbon was tested with the same procedure as used for the porous nanosheets. Dye removal tests Dye solutions (CR, MB and BY) of different concentrations were prepared by dissolving appropriate amounts of CR, MB and BY into deionised water, respectively. In a typical adsorption of CR experiment, 10 mg of the porous BN nanosheets was added to 25 ml CR aqueous solution (130 mg l −1 ) under stirring, and UV–vis absorption spectra were recorded at different time intervals to monitor the process at 496 nm. The adsorption isotherm was obtained by varying the initial CR concentration. The adsorption studies of MB and BY were similar to those of CR except for the detection wavelength difference (665 nm for MB and 412 nm for BY). The adsorption isotherms are fitted (correlation coefficients, R 2 >0.99) by using the Langmuir adsorption model [34] : Where Q e (mg g −1 ) is the amount of dyes adsorbed at equilibrium, C e (mg l −1 ) is the equilibrium solute concentration, Q m is the maximum adsorption capacity corresponding to complete monolayer coverage, and b is the equilibrium constant (l mg −1 ). How to cite this article: Lei, W. et al . Porous boron nitride nanosheets for effective water cleaning. Nat. Commun. 4:1777 doi: 10.1038/ncomms2818 (2013).